Optical separation of mechanical strain from charge doping in graphene Because of its superior stretchability, graphene exhibits rich structural deformation behaviours and its strain engineering has proven useful in modifying its electronic and magnetic properties. Despite the strain-sensitivity of the Raman G and 2D modes, the optical characterization of the native strain in graphene on silica substrates has been hampered by excess charges interfering with both modes. Here we show that the effects of strain and charges can be optically separated from each other by correlation analysis of the two modes, enabling simple quantification of both. Graphene with in-plane strain randomly occurring between −0.2% and 0.4% undergoes modest compression (−0.3%) and significant hole doping on thermal treatments. This study suggests that substrate-mediated mechanical strain is a ubiquitous phenomenon in two-dimensional materials. The proposed analysis will be of great use in characterizing graphene-based materials and devices. Since the first isolation of graphene from graphite [1] , atomically thin membranes of various materials have been studied revealing novel electronic [1] , [2] , optical [2] , [3] , chemical [4] , [5] , [6] and mechanical [7] properties distinct from those of their bulk counterparts. Many of the findings led to proposals of unique applications, for graphene in particular, such as nanoelectronics [8] , transparent conductive electrodes [9] , high-performance composites [10] , and so on. Each of the applications requires controllable modification of the material properties of graphene, for instance, electronic band gap [8] , sheet resistance [9] , or dispersibility [11] . Mechanical strain ( ) has also been predicted useful in implementing energy gaps in graphene under triangular stress [12] and confinement effects [13] like one-dimensional channels without physical cutting inducing unwanted charge localization on edges [14] . More recently, it was shown that non-uniform strain generates pseudo-magnetic field of 300 T pointing to a new application [15] . On the other hand, strain can be induced uncontrollably during various processes involved in preparation of graphene sheets and devices. In particular, thermal treatments tend to generate in-plane strain due to difference in the thermal expansion coefficients (TEC) of graphene and underlying substrates. For example, graphene epitaxially grown on SiC [16] above 1,100 °C exhibits substrate-induced compressive strain ( ~−1%) at room temperature [17] . On annealing at 300 °C, graphene on SiO 2 substrates undergoes drastic structural deformation forming sub-nm high ripples with a lateral quasi-period of several nm (ref. 4 ), implying the presence of corrugation-induced strain [18] . A similar thermal rippling was observed on a larger length scale in graphene suspended over a trench [19] . Even pristine graphene on SiO 2 substrates, prepared by mechanical exfoliation of graphite, is deformed [4] on the nm-length scale owing to the ultrastrong adhesion [20] with the undulating substrates. Although many scanning tunnelling microscopy (STM) studies have revealed corrugation [18] , [21] , [22] , [23] and related strain [18] , [23] , however, quantitative characterization of the native strain and its behaviour on thermal stress has been rare [4] , [24] . Raman spectroscopy has been a useful tool in characterizing strain in crystalline and semi-crystalline materials [25] as changes in lattice constants lead to variations in phonon frequencies. The strain-sensitivity of the Raman frequencies of G ( ω G ) and 2D ( ω 2D ) modes have been determined for graphene under uniaxial or biaxial stress by several groups with the resulting Gruneisen parameters in agreement with the theoretical predictions [26] , [27] , [28] , [29] , [30] , [31] . Both ω G and ω 2D are also strongly dependent on the extra charges induced by either electrical [32] , [33] or chemical methods [4] , [6] , [34] owing to the static effects on the bond lengths and non-adiabatic electron–phonon coupling [35] . The bimodal sensitivity of ω G and ω 2D complicates independent determination of either of strain or charge density ( n ), which typically requires prior knowledge of the other. While the wide distribution in ω G of mechanically exfoliated graphene samples were attributed to charge impurities [36] ; for instance, it is not known how much native strain contributes to the variation of ω G . Here we demonstrate that the concurrent native strain and charge doping in graphene can be determined separately from each other by Raman spectroscopy. Extensive two-dimensional Raman analysis shows that most of pristine graphene sheets exhibit strain in the range of −0.2 to 0.4%, which varies gradually on the length scale of several microns. The native strain is relieved and becomes compressive when annealed at 100 °C or above, showing rich thermal transformation behaviours. Strain- and charge-sensitivity of ω G and ω 2D First, we show that the pristine samples exhibit spatial inhomogeneity in ω G ranging from 1,573 to 1,586 cm −1 . 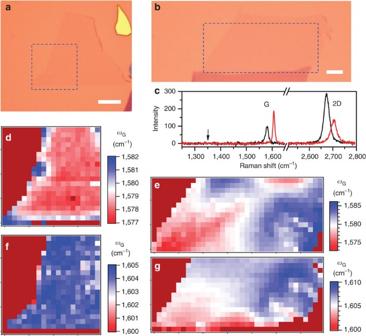Figure 1: Raman maps of single-layer graphene revealing large frequency variations. (a) Optical micrograph of sampleK1. Scale bar, 10 μm. (b) Optical micrograph of sampleK2. Scale bar, 5 μm. (c) Representative Raman spectra ofK2obtained before (black line) and after (red line) thermal annealing at 400 °C for 2 h. The absence of the disorder-related D band (marked by the vertical arrow) indicates high crystalline order of the sample. (d) Raman map for the G-mode frequency (ωG) obtained from pristineK1. (e) Raman map for the G-mode frequency (ωG) obtained from pristineK2. (f) Raman map for the G-mode frequency (ωG) obtained from annealedK1. (g) Raman map for the G-mode frequency (ωG) obtained from annealedK2. Each of the Raman mapping was carried out in the areas specified by the blue dashed boxes spanning 20×20 and 35×15 μm2forK1andK2, respectively. Each Raman spectrum of the map data was obtained for 15 s. Figure 1a,b shows optical micrographs of two graphene samples deposited on SiO 2 /Si substrates. As shown in Fig. 1c , the Raman spectra of these samples contain the two prominent peaks typifying single-layer graphene, G and 2D peaks originating from the doubly degenerate zone-centre phonon E 2g mode and overtone of the transverse optical phonon near K points in the Brillouin zone, respectively [37] . The absence of the disorder-related D peak near 1,350 cm −1 and symmetric Lorentzian line shape of the 2D peak with a width of ~25 cm −1 are the most salient features of defect-free single-layer graphene [37] . To investigate the spatial variations of the spectral features, hundreds of spectra were obtained per sample by raster-scanning the laser spot within the dashed boxes in Fig. 1a,b . The ω G -Raman maps shown in Fig. 1d,e exhibit significant random variations. Whereas the edge regions in Fig. 1d have ω G close to that of graphite (1,581.5±0.3 cm −1 ; see Methods ) with ~4 cm −1 downshift in the central region, Fig. 1e exhibits an even wider distribution over an area of 35×15 μm 2 . Besides the pixel-to-pixel variations, there are long-range undulations in ω G occurring on a length scale of several μm. We attribute most of this frequency modulation to strain as will be shown below. In addition, we found that the density of native charges in strain-dominant pristine graphene is very low (≤4×10 11 cm −2 ) when judged from various Raman spectroscopic features. (see Methods .) Figure 1: Raman maps of single-layer graphene revealing large frequency variations. ( a ) Optical micrograph of sample K1 . Scale bar, 10 μm. ( b ) Optical micrograph of sample K2 . Scale bar, 5 μm. ( c ) Representative Raman spectra of K2 obtained before (black line) and after (red line) thermal annealing at 400 °C for 2 h. The absence of the disorder-related D band (marked by the vertical arrow) indicates high crystalline order of the sample. ( d ) Raman map for the G-mode frequency ( ω G ) obtained from pristine K1 . ( e ) Raman map for the G-mode frequency ( ω G ) obtained from pristine K2 . ( f ) Raman map for the G-mode frequency ( ω G ) obtained from annealed K1 . ( g ) Raman map for the G-mode frequency ( ω G ) obtained from annealed K2 . Each of the Raman mapping was carried out in the areas specified by the blue dashed boxes spanning 20×20 and 35×15 μm 2 for K1 and K2 , respectively. Each Raman spectrum of the map data was obtained for 15 s. Full size image To investigate the effects of thermal perturbation on the native strain, the samples in Fig. 1 were annealed at 400 °C in vacuum for 2 h. The Raman spectrum obtained following the annealing reveals ~25 cm −1 increases in ω G and ω 2D ( Fig. 1c ), which occurred throughout the whole graphene sheets as shown by the ω G –Raman maps in Fig. 1f,g . The annealing-induced stiffening of both Raman modes, first reported by Li et al . [6] , was attributed to hole doping caused by O 2 in the presence of water [4] , although exact doping mechanisms still remain unclear [4] , [38] , [39] , [40] , [41] , [42] . The intensity decrease and line broadening in 2D mode of the annealed graphene ( Fig. 1c ) are also mainly attributed to the hole doping [43] , [44] . While Fig. 1f confirms the upshift in ω G across the entire area, it also reveals that the spatial variation of ω G has been removed on the annealing. On the contrary, the ω G -undulation in Fig. 1e remains almost unaffected by the thermal treatment despite the annealing-induced upshift ( Fig. 1g ). The puzzling spectral variations above are now presented in a different perspective in Fig. 2 to show how the pixel-to-pixel variations in ω G correlate with those in ω 2D . Interestingly, hundreds of data points from a given pristine sample, each corresponding to a spectral average over ~1 μm 2 , form a linear line. Remarkably, the data sets from eight pristine samples including three in Fig. 2 turned out to fall on a single line with a slope (Δ ω 2D /Δ ω G ) of 2.2±0.2 (black dashed line). To determine intrinsic frequencies of the two modes ( ω G 0 , ω 2D 0 ) not affected by strain or excess charges, we investigated a freestanding graphene ( F1 ; Supplementary Fig. S1 ) suspended across a circular well (7 μm in diameter and 5 μm in depth). The green circle in Fig. 2 indicates the values averaged over a freestanding area of 16 μm 2 , (1,581.6±0.2, 2,676.9±0.7). Freestanding graphene is known to be virtually charge-neutral with a residual charge density less than 2×10 11 cm −2 (ref. 34 ). Despite the possibility of pre-tension in the suspended graphene [45] , we conclude that F1 is essentially strain-free because ω G 0 agrees well with the aforementioned value of graphite and that of electrically neutralized bilayer graphene [46] within 0.5 cm −1 corresponding to a biaxial strain less than ~0.01% (ref. 30 ). Setting ( ω G 0 , ω 2D 0 ) as the origin ( O ) of the ω G – ω 2D space, the points near O in Fig. 2 originate from graphene areas that are nearly charge- and strain-free like the freestanding graphene and the rest are mechanically strained or charge-doped. 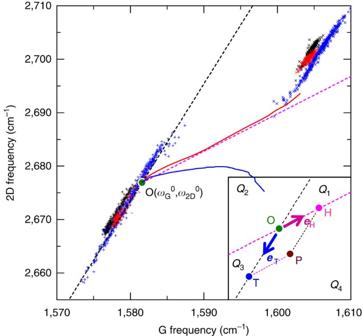Figure 2: Correlation between the frequencies of the G and 2D Raman modes of graphene (ωG,ω2D). The data were obtained from Raman mapping of three graphene samples (K1,K2andK3, respectively, in red, blue and black) before (+) and after (×) thermal annealing at 400 °C. Each Raman spectrum of the map data was obtained for 15 s. The green dot (denotedO) obtained from a freestanding graphene sample (F1) represents (ωG0,ω2D0) that is not affected by strain or charge doping. (see the text and alsoSupplementary Fig. S1) The red and blue solid lines represent (ωG,ω2D) of graphene doped with varying density of holes and electrons, respectively, induced by an electrical method (ref.49). (It is to be noted that there is an equivalent work, ref.43, which shows some discrepancy from ref.49. For detailed discussion, seeSupplementary Methods A.) The magenta dashed line is an average of experimental (ωG,ω2D) for strain-free graphene with varying density of holes (n) (refs43,49). The black dashed line represents a prediction of (ωG,ω2D) for charge-neutral graphene under randomly oriented uniaxial stress. (see the text) Inset: decomposition of the effects of hole doping and strain using a vector model. Any given (ωG,ω2D),OP, can be decomposed intoOHalong the 'strain-free' unit vector,eHfor hole doping, andOTalong the 'charge-neutral' unit vector,eTfor tensile strain (−eTfor compressive strain), respectively.eHandeTdivide theωG-ω2Dspace into the four quadrants (Q1–Q4). Figure 2: Correlation between the frequencies of the G and 2D Raman modes of graphene ( ω G , ω 2D ). The data were obtained from Raman mapping of three graphene samples ( K1 , K2 and K3 , respectively, in red, blue and black) before (+) and after (×) thermal annealing at 400 °C. Each Raman spectrum of the map data was obtained for 15 s. The green dot (denoted O ) obtained from a freestanding graphene sample ( F1 ) represents ( ω G 0 , ω 2D 0 ) that is not affected by strain or charge doping. (see the text and also Supplementary Fig. S1 ) The red and blue solid lines represent ( ω G , ω 2D ) of graphene doped with varying density of holes and electrons, respectively, induced by an electrical method (ref. 49 ). (It is to be noted that there is an equivalent work, ref. 43 , which shows some discrepancy from ref. 49 . For detailed discussion, see Supplementary Methods A .) The magenta dashed line is an average of experimental ( ω G , ω 2D ) for strain-free graphene with varying density of holes ( n ) (refs 43 , 49 ). The black dashed line represents a prediction of ( ω G , ω 2D ) for charge-neutral graphene under randomly oriented uniaxial stress. (see the text) Inset: decomposition of the effects of hole doping and strain using a vector model. Any given ( ω G , ω 2D ), OP , can be decomposed into OH along the 'strain-free' unit vector, e H for hole doping, and OT along the 'charge-neutral' unit vector, e T for tensile strain (− e T for compressive strain), respectively. e H and e T divide the ω G - ω 2D space into the four quadrants ( Q 1 – Q 4 ). Full size image Although ω G and ω 2D are highly sensitive to both n and , we note that their fractional variation due to n , (Δ ω 2D /Δ ω G ) n , is very different from that caused by , . First, biaxially strained graphene, either compressive or tensile, shows a fairly large ratio of : three groups reported experimental values of 2.45 (ref. 47 ), 2.63 (ref. 31 ), and 2.8 (ref. 30 ), whereas theory predicted slightly smaller values of 2.25 (ref. 48 ) and 2.48 (ref. 27 ). For graphene under uniaxial stress, however, depends on the direction of the strain with respect to the crystallographic axes of graphene. Because of the strain-induced symmetry breaking, the G (2D) mode of graphene under uniaxial stress splits into G − (2D − ) and G + (2D + ) [26] , [27] . When graphene is strained along the zigzag (arm-chair) directions, =2.05 (1.89) and =2.00 (3.00) [29] . When the observed G (2D) peaks are resultant of the G − (2D − ) and G + (2D + ) peaks that are not resolved because of insufficient splitting, for the zigzag (arm-chair) directions can be approximated as an average of and , 2.02 (2.44). However, as the native strain in mechanically exfoliated graphene can be aligned along any direction between the zigzag and arm-chair axes, is expected to lie in the range of 2.02–2.44, which is in an excellent agreement with 2.2±0.2 obtained from the 8 samples. Second, the effects of n are dependent on the sign of the charges because of their static effects on bond-length and are more pronounced for ω G than ω 2D because of the non-adiabatic electron–phonon coupling [32] , [33] , [35] . Hole doping induced by electrical gating leads to a quasi-linearity ((Δ ω 2D /Δ ω G ) n hole =0.75±0.04) between ω G and ω 2D as shown by the red solid line in Fig. 2 ( Supplementary Fig. S2 and Supplementary Methods A ), whereas Δ ω 2D /Δ ω G for electron doping becomes more nonlinear for high charge density as depicted by the blue solid line [49] . However, we exclude the possibility of electron-doping in the current studies because many charge transport [50] and Raman scattering [36] studies have observed hole doping predominantly in pristine [36] and annealed [4] graphene. Thus, based on the negligible charge density in these samples (Methods), we conclude that the linear variations of ω G and ω 2D are due to native strain in graphene. Although our results are in better agreement with the scenario of uniaxial strain, the presence of biaxial strain or mix of both could not be excluded viewing the disagreement in experimental and discrepancy between experiment and theory. The presence of native strain also leads to an interesting question on 'strain coherence length', how large the strained domains are or how far the direction of the strain is maintained, which is beyond the scope of the current studies. However, a recent STM study suggests that the length scale can be as small as a few nm for graphene on SiO 2 substrates [23] , which is also consistent with the spatial distribution of in-plane atomic displacements resulting from thermal fluctuation [51] . Vector decomposition of and n Now, it is logical to extract the contribution by or n for a given point in the ω G – ω 2D space, P ( ω G , ω 2D ), using a simple vector model as depicted in the inset of Fig. 2 : OP = a e T + b e H , where a and b are constants, e T and e H are unit vectors for tensile strain ( =2.2±0.2) and hole doping effects ((Δ ω 2D /Δ ω G ) n hole =0.70±0.05), respectively. The ω G – ω 2D space is now divided into four quadrants ( Q 1 – Q 4 ) by e T and e H . As increasing n ( ) of an intrinsic graphene, its values of ( ω G , ω 2D ) will move from O along e H ( e T ). Whereas Q 4 ( Q 1 ) is attributed to tensile (compressive) strain combined with hole doping, Q 2 and Q 3 are not allowed because both of electron and hole doping should lead to increase in ω G . Thus, the variations in ω G and ω 2D of the pristine graphene in Fig. 2 are mostly due to strain with negligible charge doping ( b ~0) and the extent of tensile strain is typically a few times larger than that of compressive one for a given sample. Few pristine graphene sheets of smaller area, however, exhibited non-negligible doping concurrent with strain as will be shown below. While the assumption of constant (Δ ω 2D /Δ ω G ) n hole is approximately valid on a wider frequency range, more accurate analysis of and n can be performed using a theoretical prediction [35] (blue solid line in Fig. 3 ) and the experimental data [49] for (Δ ω 2D /Δ ω G ) n hole (red solid line in Fig. 3 ) as explained below. In addition, the variation of ω G caused by the change in n , thus the Fermi level ( E F ), becomes nonlinear with respect to ΔE F at low charge density (| n |~1×10 12 cm −2 ) because of the anomalous softening [35] of G phonon occurring when ( Supplementary Methods B ). As a refined approach over the original vector model, Fig. 3a shows a new trajectory of O ( ω G 0 , ω 2D 0 ) for hole doping (blue solid line) theoretically predicted [35] by considering the phonon anomaly for n ranging from 0 to 2.6×10 12 cm −2 . With increasing n , O ( ω G 0 , ω 2D 0 ) first moves into the blue-shaded region, a forbidden area in Q 2 , and returns back into the doping-affected area ( Q 1 ) represented by the yellow shade at n ~1.4×10 12 cm −2 . As further increasing n , the refined trajectory approaches e H very closely as can be seen in Fig. 3b . In addition, the area of the blue region due to the anomalous softening (Δ ω G Anom in Fig. 3a ) is very small compared with the yellow region on a larger frequency scale as shown in Fig. 3b . We note, however, that any given point in the blue area or on the e T line, A ( ω G , ω 2D ), can be attributed to either A′ or A″ affected by strain. Thus, unambiguous determination of and n cannot be made for A in the blue shade and the associated errors turn out to be Δ ≤ 0.03% and Δ n ≤ 1.5×10 12 cm −2 . In contrast, B ( ω G , ω 2D ) in the yellow area can be unequivocally interpreted as B′ affected by compressive strain, thus enabling more accurate determination of and n . However, the experimental path (red solid line in Fig. 3a ) does not enter the blue area because of the absence of the anomalous softening of G mode as explained in Supplementary Fig. S3 . Over the wide range of n (0~1.6×10 13 cm −2 ) shown in Fig. 3b , however, the experimental (red solid line) and theoretical (blue solid line) trajectories agree well with each other and can be well represented by the e H line. Thus, the refined approach in Fig. 3b enables one to disentangle the degree of strain from that of charge doping more accurately. For the pristine graphene shown in Fig. 3b , for example, it can be seen that ranges from −0.2 to 0.4% with n <1.0×10 12 cm −2 for the majority of the data points. It should be noted, however, that few experimental data sets [43] , [49] for (Δ ω 2D /Δ ω G ) n hole available in the literature reveal non-negligible discrepancy ( Supplementary Fig. S3 ) and thus refined experimental data will enhance the accuracy of the proposed analysis. 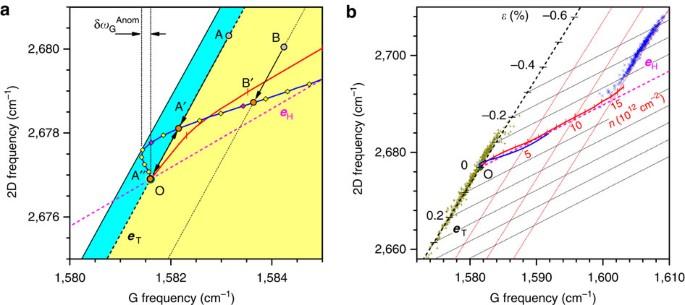Figure 3: Refined analysis model considering the logarithmic phonon anomaly. (a) The effects of hole carriers with varying densitynon (ωG,ω2D) of graphene. The red solid line presents the experimental trajectory of (ωG,ω2D) as a function ofnobtained by Daset al. (ref.49). The red vertical bars on the red solid line markn, every 1.0×1012cm−2. The blue solid line represents a theoretical prediction by Lazzeriet al. reported in ref.35that considered the effects of the logarithmic phonon anomaly. We used the relationship thatωG(n)=ωGo+ΔωG(n) andω2D(n)=ω2Do+Δω2D(n), where (ωGo,ω2Do) corresponds toOofFig. 2. The numerical values of Δω2D(n) were obtained assuming its linear relationship with ΔωG(n) as shown inSupplementary Fig. S3b. The hole density (n) for the blue solid line ranges from 0 (corresponding toO) to ~2.6×1012cm−2as marked by the yellow and magenta diamonds every 0.2×1012and 1.0×1012cm−2, respectively. (b) The theoretical and experimental trajectories of (ωG,ω2D) affected bynranging from 0 to 1.6×1013cm−2with Raman map data of pristine (+) and annealed (×)K2. The red solid line is identical to the one ina. The black horizontal bars on theeTline designate uniaxial strain () ranging from −0.6 to 0.3%, each bar representing a step of 0.1%. The uniaxial strain-sensitivity of the G mode, ΔωG/Δ=−23.5 cm−1/%, was calculated from the work by Yoonet al. (ref.29) considering the splitting of the G mode and random crystallographic orientation of strain. In case of biaxial strain, however, an averaged sensitivity factor of −69.1±3.4 cm−1/% can be used (refs27,30,47). Figure 3: Refined analysis model considering the logarithmic phonon anomaly. ( a ) The effects of hole carriers with varying density n on ( ω G , ω 2D ) of graphene. The red solid line presents the experimental trajectory of ( ω G , ω 2D ) as a function of n obtained by Das et al . (ref. 49 ). The red vertical bars on the red solid line mark n , every 1.0×10 12 cm −2 . The blue solid line represents a theoretical prediction by Lazzeri et al . reported in ref. 35 that considered the effects of the logarithmic phonon anomaly. We used the relationship that ω G ( n )= ω G o +Δ ω G ( n ) and ω 2D ( n )= ω 2D o +Δ ω 2D ( n ), where ( ω G o , ω 2D o ) corresponds to O of Fig. 2 . The numerical values of Δ ω 2D ( n ) were obtained assuming its linear relationship with Δ ω G ( n ) as shown in Supplementary Fig. S3b . The hole density ( n ) for the blue solid line ranges from 0 (corresponding to O ) to ~2.6×10 12 cm −2 as marked by the yellow and magenta diamonds every 0.2×10 12 and 1.0×10 12 cm −2 , respectively. ( b ) The theoretical and experimental trajectories of ( ω G , ω 2D ) affected by n ranging from 0 to 1.6×10 13 cm −2 with Raman map data of pristine (+) and annealed (×) K2 . The red solid line is identical to the one in a . The black horizontal bars on the e T line designate uniaxial strain ( ) ranging from −0.6 to 0.3%, each bar representing a step of 0.1%. The uniaxial strain-sensitivity of the G mode, Δ ω G /Δ =−23.5 cm −1 /%, was calculated from the work by Yoon et al . (ref. 29 ) considering the splitting of the G mode and random crystallographic orientation of strain. In case of biaxial strain, however, an averaged sensitivity factor of −69.1±3.4 cm −1 /% can be used (refs 27 , 30 , 47 ). Full size image Thermal modulation of and n We demonstrate that thermal annealing in vacuum removes the native tensile strain and induces compressive strain. The most prominent change caused by the thermal annealing in Fig. 2 is that the concurrent stiffening of the G and 2D modes. The refined analysis model in Fig. 3b readily leads to quantification of strain and charge density: despite the wide distribution, most of the ( ω G , ω 2D ) points of annealed K2 lie on a line parallel to e T with ~80% of the thermally induced changes in ω G found along the e H axis. This indicates that the O 2 -induced hole doping activated by annealing [4] dominates the spectral changes and n remains relatively constant at (1.4±0.1)×10 13 cm −2 . The wide distributions in ω G and ω 2D , instead, can be attributed to compressive strain (−0.3% ≤ ≤ 0), which contrasts with the fact that the native strain was mostly tensile in nature. This finding is in agreement with the annealing-induced slippage [19] , [24] and buckling [4] of graphene on SiO 2 substrates caused by the difference in TECs of both materials [52] , because the former relieves the tensile stress [24] and the latter accompanies compression [19] . We also note that thermal modulation of strain is sample-specific. For example, the spectral spreads of K1 and K3 in the ω G – ω 2D space decreased greatly on annealing, while those of K2 underwent only minor changes as shown in Fig. 2 . Presenting the ω G − ω 2D graph obtained from K4 in Fig. 4 , we varied the annealing temperature stepwise to determine the critical temperatures where the native strain starts to relax and changes into compression. It can be seen that the pristine graphene has mostly tensile strain with negligible hole doping: each P ( ω G , ω 2D ) of K4 lies on the e T axis in the range between (1,578, 2,670) and (1,582, 2,678). Following the first annealing at 100 °C, most of P ( ω G , ω 2D ) moved into the range between (1,580, 2,676) and (1,585, 2,683), but still mostly along e T . This change demonstrates that heating at 100 °C can be sufficient to remove most of the native tensile strain and compress graphene, simultaneously causing slight hole doping at certain areas. Although subsequent annealing at 150 °C led to more obvious hole doping in addition to further compression, repeated annealing at 200, 250 and 300 °C resulted in less significant variations in P ( ω G , ω 2D ); data for the treatments at 200 and 250 °C are not shown to avoid congestion. Further treatments at 400 and 500 °C, however, induced marked movement of P ( ω G , ω 2D ) to (1,591.5±1.4, 2,693±2.3) and (1,598.4±1.4, 2,698±2.6), respectively. The changes are largely in parallel with e H , indicating emergence of strong hole doping. 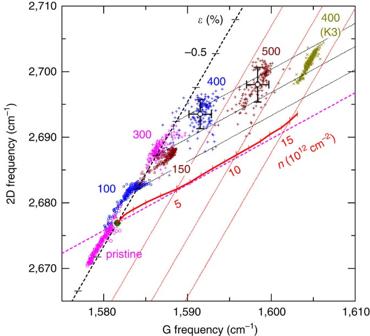Figure 4: Thermally induced variations in (ωG,ω2D) on successive annealing. The data were obtained from Raman mapping of a graphene sample (K4) before and after successive thermal annealing at various temperatures (Tannealin °C), except those in dark yellow that were obtained fromK3following the one-time annealing at 400 °C (seeFig. 2). The horizontal and vertical error bars forTanneal=400 & 500 °C represent s.d. inωGandω2D, respectively. Each Raman spectrum of the map data was obtained for 10 s. Figure 4: Thermally induced variations in ( ω G , ω 2D ) on successive annealing. The data were obtained from Raman mapping of a graphene sample ( K4 ) before and after successive thermal annealing at various temperatures ( T anneal in °C), except those in dark yellow that were obtained from K3 following the one-time annealing at 400 °C (see Fig. 2 ). The horizontal and vertical error bars for T anneal =400 & 500 °C represent s.d. in ω G and ω 2D , respectively. Each Raman spectrum of the map data was obtained for 10 s. Full size image We also note hysteretic effects in annealed graphene samples. Compared with the one-time annealing at 400 °C ( K1 – K3 in Fig. 2 ), the sample ( K4 ) that underwent cycles of prior annealing at lower temperatures exhibit much less changes but larger distributions in frequencies ( Fig. 4 ) and linewidths ( Supplementary Fig. S4 ). As the buckling of annealed graphene sheets responsible for the thermally induced hole doping [4] is dictated by adhesion and slippage of graphene on silica [19] , [24] , it is likely that prior history of thermal treatments affects the buckling behaviours and thus ω G and ω 2D . The spectral inhomogeneity increased by the repeated annealing cycles can be attributed to further structural deformation or in - situ reactions with residual gases in the vacuum system during annealing or post-annealing surface reactions [6] occurring in the ambient conditions. As annealing is widely used in fabricating graphene transistors [50] and preparing graphene samples for various fundamental research [18] , [21] , the exact chemical changes made by annealing deserve careful studies in the future. The Lorentzian linewidths of G ( Γ G ) and 2D ( Γ 2D ) peaks, and the 2D/G peak area ratios ( A 2D / A G ), determined following each annealing cycle, are also consistent with the scenario of thermally induced mechanical transformation concurrent with hole doping ( Supplementary Fig. S4 and Supplementary Methods C ). Spatial mapping of and n In Fig. 5 , we demonstrate that the native strain concurrent with spatially varying charge doping can be optically mapped out using the refined vector analysis. The Raman maps obtained from the graphene sample ( K5 in Fig. 5a ) reveal that ω G , ω 2D and Γ G exhibit variations of several cm −1 across an area of 20×15 μm 2 , respectively, in Fig. 5b–d . Unlike the strain-dominated graphene ( K1 – K4 ), all P ( ω G , ω 2D ) from K5 are scattered in Q 4 instead of forming a line along e T ( Fig. 5g ), indicating the coexistence of tensile strain and hole doping. According to the vector analysis in Fig. 2 , each point of P ( ω G , ω 2D ) can then be decomposed into and T ( ω G , ω 2D ) n =0 , representing phonon frequencies which are not affected by or n , respectively. Shown in Fig. 5e,f are the resulting Raman maps of and ω G, n =0 : resorting to Fig. 5g ; the former reveals the spatial distribution of the hole density ranging up to 3.5×10 12 cm −2 , whereas the latter maps out the native strain (−0.03%< <0.17%). Fig. 5e,f also reveal that the long-range distribution of the strain does not necessarily coincide with the native charge distribution. It is also to be noted that and Γ G obey a reciprocal relation that conforms to the theoretical prediction for charge doping [43] , whereas ω G and Γ G exhibit a much broader distribution due to the coexisting strain ( Supplementary Fig. S5 ). Similar improvement was obtained in the correlation between and A 2D / A G ( Supplementary Fig. S5 ). 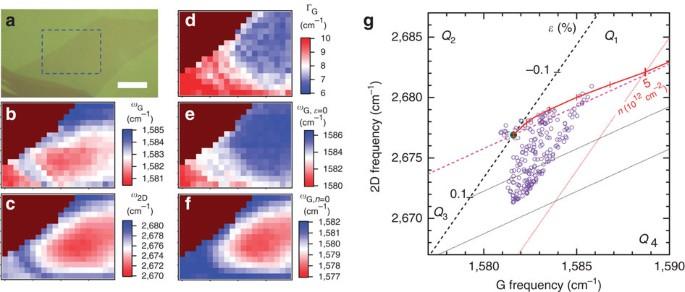Figure 5: Decomposition of the effects of strain concurrent with spatially varying charge doping in pristine graphene. (a) Optical micrograph of a graphene sample (K5) under tensile stress concurrent with charge doping. Scale bar, 10 μm. (b) Raman map ofωG. (c) Raman map ofω2D. (d) Raman map forΓG. (e) Raman map of. (f) Raman map ofωG,n=0. (g) Correlation betweenωGandω2Dthat were given inbandc. The Raman map data ina–cwere obtained from pristineK5for 10 s/pixel from the area (20×15 μm2) indicated by the blue dashed box ina. The data ineandfwere mathematically derived by the simple vector model described inFig. 2(see the text). Figure 5: Decomposition of the effects of strain concurrent with spatially varying charge doping in pristine graphene. ( a ) Optical micrograph of a graphene sample ( K5 ) under tensile stress concurrent with charge doping. Scale bar, 10 μm. ( b ) Raman map of ω G . ( c ) Raman map of ω 2D . ( d ) Raman map for Γ G . ( e ) Raman map of . ( f ) Raman map of ω G, n =0 . ( g ) Correlation between ω G and ω 2D that were given in b and c . The Raman map data in a – c were obtained from pristine K5 for 10 s/pixel from the area (20×15 μm 2 ) indicated by the blue dashed box in a . The data in e and f were mathematically derived by the simple vector model described in Fig. 2 (see the text). Full size image The current study shows that most of graphene on silica substrates are mechanically strained and tensile strain is more frequently found than compressive one in a given sample. In this regard, graphene can be envisaged as food wrap that tends to become strained forming ripples when clinging to flat surfaces. Although both tensile and compressive shear stresses can be applied to the membrane, facile buckling along the out-of-plane direction will make compressive strain less likely than tensile one. Interestingly, the extent of the native strain is the larger on average for the larger graphene flake, which may be due to the fact that larger contact area with substrates provides enhanced adhesion to resist slippage caused by in-plane stress. However, thermal perturbation as shown in the current study and varying interactions with other substrates should lead to diverse structural transformation of graphene and other newly discovered two-dimensional materials such as h -BN, MoS 2 , MoSe 2 , and so on. We also note that strain dominates the spectral variations over charge doping that has been considered mainly responsible for the spectral irregularities in graphene [36] . This suggests that the degree of mechanical deformation or charge doping depends on preparation methods. Insignificant chemical doping in our pristine samples could be due to different chemical and structural properties of the substrate surfaces [38] . In this regard, the presence of tensile strain in graphene may have an influence on the degree of charge doping. A recent STM study revealed that graphene is partly suspended between microscopic hills of the substrates when supported on SiO 2 substrates [22] . Tensile stress is likely to induce localized suspension of graphene that otherwise would largely conform [18] to the undulating substrates owing to the van der Waals interaction [20] . ( Supplementary Methods D .) Such semi-freestanding graphene should be less sensitive to charge-doping that occurs via contact with the substrates [34] , [38] , [40] or through the corrugation-mediated mechanisms [4] , [6] . We also note that strain may give rise to charge inhomogeneity through rehybridization of π–σ bonds and vice versa [53] , [54] . However, no clear correlation was found as shown in Figs 1 and 5 and Methods, presumably, because of the insufficient spatial resolution and limited sensitivity towards charge density and strain. The spatial distribution of native strain in mechanically exfoliated graphene samples has rarely been quantified [23] . Moreover, the strain has not been systematically considered in interpreting Raman spectra owing to the competing effects of extra charges, despite the well-characterized strain-sensitivities of the G and 2D bands [26] , [27] , [28] , [29] , [30] , [31] . Our studies demonstrate that the G and 2D Raman modes of graphene can be highly reliable in determining mechanical strain and charge density even when both coexist. The bimodal sensitivity of both modes, however, requires careful interpretation as suggested in this paper. Although many STM studies revealed structural irregularities such as buckling and strain in graphene [18] , [21] , [22] , [23] , the method is not practically useful in achieving statistical information on a length scale larger than microns. Moreover, the current studies demonstrate that graphene undergoes sample-specific hysteretic structural deformation on thermal treatments and possibly other external perturbations. As typical microfabrication [50] and STM measurements [18] , [21] of graphene and its devices involve various sample treatments such as annealing, transfer to substrates, polymer coating, wetting-drying, and so on., their effects need be considered in interpreting results. Our studies also suggest that not only graphene but also other two-dimensional materials supported on solid substrates are generally susceptible to native strain and thermal deformation owing to zero-dimension along the z axis and different TECs of involved materials. Despite providing a systematic analysis, however, the current study also shows some limitations. In principle, simultaneous vector decomposition into strain, p -type, and n -type doping cannot be made unambiguously requiring that contribution of at least one component should be known or assumed. The non-zero dispersion of ω 2D limits the current approach to the Raman measurement obtained with 514 nm as an excitation source. Follow-up studies are being carried out with other excitation wavelengths. This work is also limited to single-layer graphene, and analysis of few-layer graphene will require separate set of data. Finally, the accuracy of this approach will be directly affected by the spectral accuracy of employed spectrometers that can be tested against O ( ω G 0 ω 2D 0 ). In conclusion, we have demonstrated that the native strain can be unambiguously determined by Raman spectroscopic analysis notwithstanding the interference from the coexisting charge-doping effects. Most of the pristine graphene sheets deposited onto SiO 2 substrates, by the mechanical exfoliation method, were shown to be under in-plane stress with the resulting strain in the range of −0.2~0.4%. The native tensile strain was relieved by thermal annealing at a temperature as low as 100 °C and converted to compressive strain by annealing at higher temperatures, which also induced strong hole doping clearly resolved in the analysis. The proposed analysis should be useful for fast and reliable characterization of strain and excess charges in graphene materials and devices. Preparation and treatment of samples High-quality graphene samples were prepared by the micromechanical exfoliation method [50] using kish graphite (Covalent Materials) and adhesive tape (3 M). The Si substrates with 285-nm-thick SiO 2 layers were cleaned with piranha solutions before the deposition of graphene. For freestanding graphene samples, substrates with micron-scale circular wells (diameter: 2–7 μm, depth: 5 μm) were employed [45] . For thermal annealing, samples in a tube furnace evacuated to a pressure of 3 mTorr were heated to a target temperature ( T anneal ) within 30 min, maintained at T anneal for 2 h, and then cooled down to 23 °C for ~3 h. Raman spectroscopy The number of layers and crystallinity of the prepared samples were characterized by Raman spectroscopy [37] . All the Raman spectra were obtained in a backscattering geometry using a X40 objective lens (numerical aperture=0.60) in the ambient conditions. An Ar ion laser operated at a wavelength of 514.5 nm was used as an excitation source. Whereas the spectral width of the instrument response function was determined to be 3.0 cm −1 from the Rayleigh scattering peak, the spectral precision and accuracy were better than 1.0 cm −1 from repeated measurements of Raman standards. (see below for detailed analysis.) For two-dimensional Raman maps, spectra were obtained every 1 μm using an x – y motorized stage. The average power of the excitation laser beam was 1.5 mW that was focussed onto a spot of ~0.5 μm in diameter. No irreversible photoinduced change was detected during the measurements. Spectral accuracy of the Raman measurements Although single-grating spectrometers of Czerny–Turner type, including the one (SP2300, Princeton Instruments) employed in the current study, provide high throughput and small footprints [55] , careful calibration is required to achieve instrument-limited spectral accuracy because of the wavelength dependence of its reciprocal linear dispersion [56] . More specifically, wavelength ( λ ) of each charge-coupled device detector pixel needs to be expanded in series of the pixel position ( x ): λ=λ 0 +a 1 ( x − x 0 )+a 2 ( x − x 0 ) 2 +a 3 ( x − x 0 ) 3 +...+a n ( x − x 0 ) n , where a n , λ 0 and x 0 are constants, the centre wavelength and its position on the detectors, respectively. Supplementary Fig. S6a presents the wavelengths of 13 plasma lines from the Ar laser and 3 Hg atomic lines as a function of their pixel positions recorded in the charge-coupled device detector. Although the data seem to be well described by the linear line in blue, the first order calibration with a n =0 (n > 1) leads to non-negligible error of −0.15~0.25 nm in wavelength as can be seen in Supplementary Fig. S6b . We note that this amount of deviation translates into Raman shift error of 5.0~−6.8 cm −1 that is even larger than the linewidth of the Rayleigh line (3.0 cm −1 ). It is also to be noted that a first order calibration using only 3 Hg lines (546.075, 576.961 & 579.067 nm) instead of the above 16 lines generates even larger error up to 0.68 nm or 18 cm −1 across the entire detector area. When the quadratic term was included in the calibration as shown in Supplementary Fig. S6b , however, the deviation remained within ±0.01 nm or ±0.3 cm −1 , which is sufficient in accuracy for the employed spectrograph with a focal length of 300 mm and a grating with 1,200 grooves mm −1 . This suggests that extra caution needs to be paid when comparing Raman G and 2D frequencies recorded by different spectrographs with modest spectral resolving power. We further tested the accuracy by measuring the G band frequency ( ω G ) of thick graphite flakes: ω G from 12 different spots out of four different samples was 1,581.5±0.3 cm −1 , which turned out to be within ~0.5 cm −1 from the literature values of 1,581–1,582 cm −1 (refs 57 , 58 ). Thus, the accuracy of our measurements was conservatively claimed as 1.0 cm −1 . Negligible native charge density in pristine graphene The scheme of vector decomposition proposed in this article assumes that the variation in ( ω G , ω 2D ) of the employed pristine samples except K5 is mostly due to strain and that the contribution of charge doping is sufficiently small for graphene under tensile stress. This hypothesis is well supported by a few different spectral features of the pristine samples as shown below. Supplementary Figure S7a shows that ( ω G , ω 2D ) of the three samples lies on the black-dashed line ( e T ) representing graphene affected by strain, but not charge. Moreover, the 2D/G peak area ratio ( A 2D / A G =5.8±0.3) in Supplementary Fig. S7b remains constant and very close to that ( A 2D / A G 0 =6.2±0.2) of the charge-neutral freestanding sample ( F1 ) while ω 2D varies by more than 10 cm −1 . (see Supplementary Methods E for the optical artefact caused by the substrates that affects the apparent A 2D / A G .) As A 2D / A G decreases drastically as increasing the charge density ( n ) for either type of charges [43] , Supplementary Fig. S7b supports that the presented pristine graphene samples have negligible charge density regardless of the widely varying native strain. The behaviour of Γ G that is not affected by the optical artefact will be useful in judging the native charge density. As shown in Supplementary Fig. S7c , Γ G of the three pristine samples lies in the range of 13.1±0.7 cm −1 , which is only slightly smaller than that of the freestanding sample, Γ G 0 =13.9±0.2 cm −1 . As Γ G is sensitive to low level of charge doping owing to the blockage of the non-adiabatic decay channel of the G phonon, the native charge density in the pristine samples are generally very small [34] . A quantitative estimation of n according to the model proposed by Berciaud et al . [34] leads to a conclusion that Γ G =13.1±0.7 cm −1 translates into | n |<4×10 11 cm −2 . (equation (1) and Supplementary Fig. S4 of ref. 34 were employed.) This level of charge density is an order of magnitude lower than the variations reported for graphene supported on SiO 2 substrates by others [34] , [36] . The distribution of Γ 2D as a function of ω 2D shown in Supplementary Fig. S7d also supports the assumption that the pristine graphene samples of which ( ω G , ω 2D ) lies on e T in Supplementary Fig. S7a are not affected by significant level of charge doping. Das et al . [43] showed that Γ 2D increases by ~30% in contrast to decreasing Γ G when | n | is raised to ~2×10 13 cm −2 by an electrical method. Several groups reported that Γ 2D of supported graphene samples with some level of p-type doping lies in the range of 28–30 cm −1 (refs 36 , 59 ), which is significantly larger than that of freestanding graphene (22.5–24 cm −1 ) [34] . We confirmed that Γ 2D of the charge neutral freestanding graphene ( F1 ) is 23.1±0.2 cm −1 , and found that Γ 2D of the supported samples in Supplementary Fig. S7d also remains at very small values, 23.5±1.2 cm −1 , indicating low level of native charge density. How to cite this article: Lee, J. E. et al . Optical separation of mechanical strain from charge doping in graphene. Nat. Commun. 3:1024 doi: 10.1038/ncomms2022 (2012).